Experimental drying intensifies burning and carbon losses in a northern peatland For millennia, peatlands have served as an important sink for atmospheric CO 2 and today represent a large soil carbon reservoir. While recent land use and wildfires have reduced carbon sequestration in tropical peatlands, the influence of disturbance on boreal peatlands is uncertain, yet it is important for predicting the fate of northern high-latitude carbon reserves. Here we quantify rates of organic matter storage and combustion losses in a boreal peatland subjected to long-term experimental drainage, a portion of which subsequently burned during a wildfire. We show that drainage doubled rates of organic matter accumulation in the soils of unburned plots. However, drainage also increased carbon losses during wildfire ninefold to 16.8±0.2 kg C m −2 , equivalent to a loss of more than 450 years of peat accumulation. Interactions between peatland drainage and fire are likely to cause long-term carbon emissions to far exceed rates of carbon uptake, diminishing the northern peatland carbon sink. Over the past decade, peat fires have emerged as an important issue to human health, economic loss and global climate change [1] , [2] , [3] . Land use change in tropical peatlands has lowered water table position and increased fire severity, leading to carbon losses equivalent to as much as 40% of global fossil fuel combustion in some years [1] . More than 90% of the world's peatlands, however, are found in high-latitude regions [4] , where they also are vulnerable to large wildfires [5] . Burning of disturbed peatlands is thought to have been a major contributor to the large wildfires that affected Russia in 2010, causing as much as US$15 billion in damages, and reduced industrial output [6] , [7] . Yet, no studies have investigated the influence of lowered water table position on the vulnerability of northern peatlands to burning. In 2001, a long-term peatland drainage experiment in Canada [8] burned during a wildfire, allowing us to examine the effects of two decades of drainage on fire severity and carbon losses in a boreal peatland. Peatlands accumulate peat due to positive net ecosystem carbon balance, where net primary productivity exceeds decomposition and other soil carbon losses. Because of carbon storage in peat, northern peatlands currently have a net cooling effect on climate radiative forcing [9] . However, changes in either long-term carbon uptake or losses resulting from changes in climate or land use could alter the function of peatlands within the climate system. Across the boreal region, peatland hydrology is affected by numerous land uses, including drainage for agriculture, forestry, peat harvesting, and oil and gas extraction [10] , [11] , [12] , [13] . Agriculture and forestry are considered the primary land uses affecting peatlands globally. These activities have affected about 400,000 km 2 of extratropical peatlands, equivalent to 12% of the 3.46×10 6 km 2 of boreal and subarctic peatland [13] . Linear features such as roads and seismic lines also impede peatland hydrology [14] , and are found at densities of 1.8 km km −2 in northern Alberta [15] . If current economic practices are continued, linear features in this region are expected to reach 8 km km −2 by the next century [15] , probably becoming a dominant land use change affecting Canadian peatlands. In addition to changes in land use practices, warming and increased evapotranspiration associated with climate change will lead to drying of peatlands unless increases in precipitation alleviate soil moisture deficits [16] , [17] . Whereas projected annual water yields in North American basins vary by region and by global or regional climate model scenarios, higher evapotranspiration from warming generally is expected to compensate for increases in precipitation in some regions and will magnify the effects of precipitation declines in other regions [18] , [19] . Boreal ecosystems in particular are estimated to have a high potential vulnerability to climate change in the long term [20] . Summer daily mean temperatures in Canada's boreal region are predicted to warm by 1.5–2.5 °C. Whereas precipitation is expected to increase by ∼ 20% in eastern Canada, precipitation is not expected to increase in western regions [18] , [21] where peatlands are most likely to burn [5] , [22] . Across Canada's boreal region, warming is widely expected to result in declining soil moisture and a significant increase in the frequency of large fires [21] . Similar climate-related drying is expected in Russia, with increased drought, length of fire season, and area of fire risk in the southern forest zone boundary [23] . The combined effects of changing land use and climate present substantial risks to boreal peatlands. Here we capitalize on a unique long-term experiment to examine changes in tree productivity and soil organic matter accumulation across a factorial combination of burning and drainage in a peatland in boreal western Canada. We show that a decline in the water table stimulated tree productivity and organic matter accumulation in soils, but also changed the conditions for wildfires such that combustion of soil organic matter increased ninefold, leading to large losses of carbon from the peatland. Effects of drainage on tree productivity and soil organic matter accumulation Fens represent more than 60% of total peatland cover in western Canada, where peatlands typically have a well-established tree or shrub layer [24] . In 1983, a large portion of a boreal treed fen in western Canada was experimentally drained as part of the Alberta wetlands drainage and improvement program [8] ( Fig. 1 ). In the experiment, water table position was immediately lowered by about 25 cm via drainage of the fen [14] . However, hydrologic impacts diminished over time as trenches infilled, resulting in a difference in water table position between drained and pristine (undrained) portions of the fen averaging 10 cm in 2003. In 2001, a 105,000 ha wildfire burned part of the fen complex, impacting a portion of both the experimentally drained and pristine areas. 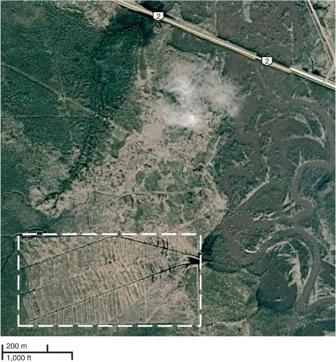Figure 1: Large-scale experimental drainage in a boreal fen. Aerial image of drainage trenches (outlined in dashed white line) in a boreal peatland in Alberta, Canada. ©2011 Google-Imagery ©2011DigitalGlobe, Cnes/Spot Image, GeoEye, Map data. Figure 1: Large-scale experimental drainage in a boreal fen. Aerial image of drainage trenches (outlined in dashed white line) in a boreal peatland in Alberta, Canada. ©2011 Google-Imagery ©2011DigitalGlobe, Cnes/Spot Image, GeoEye, Map data. Full size image Two years post-fire, we established replicate plots along a factorial combination of drainage (drained versus pristine) and burning (burned versus unburned). In the unburned plots, annual tree-ring widths were similar across the plots before drainage ( Fig. 2 ). From 1950 to 1980 (that is, pre-drainage), there was no difference in average tree-ring widths, which were 0.59±0.08 and 0.58±0.09 mm in the drained and pristine plots, respectively. In the pristine plots, ring widths increased slightly around 1993 but progressively declined through the 2000s back to this multi-decadal average. This pattern also was observed in the drained plots, but was overwhelmed by a large increase in ring width after 1986, presumably following a several year, post-drainage lag. Ring widths in the drained plots declined after 2001, possibly indicative of a longer term trend of declining tree productivity associated with reduced nutrient availability and/or in-filling of the drainage trenches. 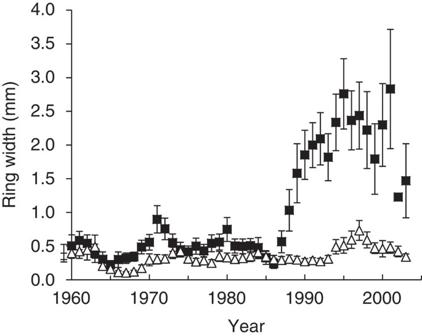Figure 2: Drainage of a boreal fen increased tree productivity. Annual changes in tree ring width in unburned pristine and drained plots. Solid squares represent data from plots that were drained in 1983. Open triangles represent data from the pristine (undrained) plots. Data are means±one standard error of multiple basal tree disks collected within the pristine and drained plots. Figure 2: Drainage of a boreal fen increased tree productivity. Annual changes in tree ring width in unburned pristine and drained plots. Solid squares represent data from plots that were drained in 1983. Open triangles represent data from the pristine (undrained) plots. Data are means±one standard error of multiple basal tree disks collected within the pristine and drained plots. Full size image Radiocarbon dating of replicate peat cores showed greater organic matter accumulation rates in the drained plots than in pristine plots. Vertical organic matter accumulation rates averaged 0.07±0.03 and 0.16±0.06 cm peryear in the pristine and drained plots, respectively ( Table 1 ). Bulk density also was higher in peat from the drained plots relative to the pristine plots ( Fig. 3 ). Because of faster vertical accumulation rates and the accumulation of denser peat, carbon accumulation rates in the drained plots (68.7±15.1 g C m −2 yr −1 ) were twice as those in the pristine plots (33.9±10.8 g C m −2 yr −1 ). Table 1 Results of radiocarbon dating and corresponding peat carbon accumulation rates across the unburned pristine (undrained) and drained plots. 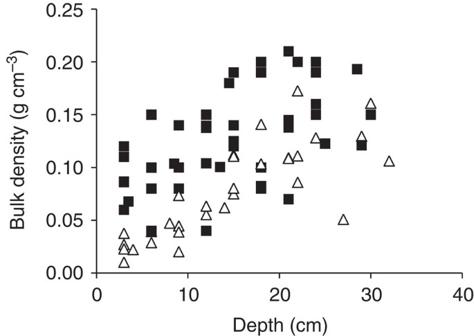Figure 3: Long-term drainage led to the formation of dense surface soils. Relationships between soil bulk density and depth in unburned pristine and unburned drained plots. Solid squares represent data from the drained plots, while open triangles represent data from the pristine plots. Full size table Figure 3: Long-term drainage led to the formation of dense surface soils. Relationships between soil bulk density and depth in unburned pristine and unburned drained plots. Solid squares represent data from the drained plots, while open triangles represent data from the pristine plots. Full size image Effects of drainage on ground fuel combustion In northern forests and peatlands, the upper few cm of live moss and vascular litter, as well as the underlying peat (that is, ground fuels, collectively), are vulnerable to burning and represent more than 85% of the total fuels consumed during Canadian forest fires [25] . In our pristine plots, the depth of combustion losses of ground fuel averaged 7±1 cm, but increased to 19±3 cm in drained plots ( Fig. 4 ). Distributions of soil carbon content with depth were used to calculate carbon losses from the depth of burn measurements. Carbon losses due to burning in the pristine plots averaged 2.0±0.5 kg C m −2 . However, carbon losses from the drained plots were approximately ninefold higher, averaging 16.8±0.2 kg C m −2 . 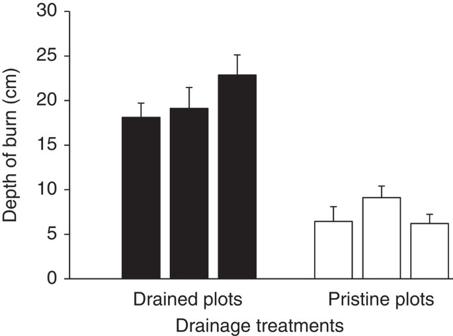Figure 4: Effects of experimental drainage on depth of ground fuel combustion. More canopy fuels in combination with drier, denser ground fuels in the drained plots probably contributed to the large combustion losses during wildfire. Data are means±one standard error of depth of burn measurements collected in replicate burned pristine (undrained) and drained plots. Figure 4: Effects of experimental drainage on depth of ground fuel combustion. More canopy fuels in combination with drier, denser ground fuels in the drained plots probably contributed to the large combustion losses during wildfire. Data are means±one standard error of depth of burn measurements collected in replicate burned pristine (undrained) and drained plots. Full size image Our results show that 20 years of experimental drainage doubled rates of carbon accumulation in soils in a fen complex, relative to pristine, undrained areas of the same complex. These results are surprising, because a lower water table position generally is expected to stimulate microbial decomposition of soil organic matter [26] . Although we did not measure decomposition rates, it is possible that microbial activity is greater in the more oxic soils of the drained plots relative to the pristine plots. However, rates of peat accumulation also are dependent on carbon inputs to soils. Others also have found that long-term drainage can stimulate above- and below-ground tree productivity, and soil carbon sequestration as silvic peat [27] , [28] , [29] . In part because of increases in tree productivity, the drainage of Finnish peatlands reduced radiative forcing by ∼ 3 mW m −2 (ref. 28 ). In some boreal regions, then, the sustained drying or drainage of peatlands in the absence of wildfire could have a negative feedback to climate change, at least in the short term, although reduced carbon uptake by trees as stands mature could diminish this effect [28] . Wildfire generally is regarded as the most important stand-replacing disturbance in the boreal biome. Yet, only a few studies have quantified combustion losses in pristine northern peatlands [30] , [31] , [32] . Previous studies have shown that depth of burn is primarily controlled by fire weather, soil moisture and seasonal ice conditions, as well as fuel bulk density [30] , [31] , [33] . In general, the combustion values measured in our pristine plots (2.0±0.5 kg C m −2 ) were consistent with these previous studies, in which combustion rates averaged 2.4 kg C m −2 . During the 1997 El Niño event, severe burning of disturbed peat in Indonesia emitted an average of 31.5 kg C m −2 (ref. 1 ). Here we describe extreme burning of boreal peat that has been triggered by decreased water table position sustained over 20 years, with carbon emissions (16.8±0.2 kg C m −2 ) more comparable to the 1997 tropical fires. We quantified carbon losses associated with the burning of ground fuels only. Combustion of above ground fuels also was probably greater in the drained plots, given an increase in canopy fuel loading from increased tree productivity and biomass. Interestingly, our results show some indication of declining tree growth in the drained plots, suggesting that tree productivity in the drained plots eventually could be constrained by nutrient availability. However, these results also could reflect changes in water table associated with in-filling of the drainage trenches over time. Though organic matter accumulation increased following drainage, severe burning in the drained plots triggered the complete loss of this carbon pool sequestered post-drainage, plus a further ∼ 450 years worth of peat accumulation (relative to 58 years of peat accumulation combusted in the pristine plots). With a regional peatland fire return interval of ∼ 120 years [5] , the combustion of old carbon in deeper peat layers suggests that fire-induced carbon losses in drained peatlands would far exceed carbon uptake between fire events. Currently, an average of 1,850 km 2 of peatland burns annually in western Canada [5] , but the annual area burned across boreal Canada is expected to increase by 200–300% over the next 50–100 years [34] . This study suggests that natural or anthropogenic declines in the water table of northern peatlands not only can stimulate short-term rates of carbon accumulation in both above- and below-ground pools, but also change the conditions for wildfires such that these enhanced carbon stores, plus a large amount of older soil carbon, become vulnerable to burning and release to the atmosphere. Climate change and land use clearly can influence peatland water tables, but whether these changes will have positive or negative consequences for net ecosystem productivity and long-term soil carbon storage will depend on interactions with periodic fire events. Results from this study document significant combustion losses of soil carbon due to interactions between fire and land use at rates that could make northern peatlands a large carbon source in the future. Description of study site The experimental fen is located 36 km southeast of Slave Lake, Alberta at 55°10′N, 114°15′W. The site is a moderate rich fen and, before drainage, was dominated by Picea mariana , Larix laricina , Betula glandulosa , Drepanocladus and Sphagnum spp [8] , [35] . Maximum peat depth at the site was 4 m (ref. 35 ), which is typical of western Canadian peatlands. The site was partially burned in a wildfire (LWF-063), which ignited on May 23, 2001 near the town of Chisholm, Alberta and burned 105,000 ha over a period of 27 days. Although considered a major fire event, this fire is not atypical of periodic large fires in this region that occur on a roughly decadal cycle. Burning caused complete tree mortality in portions of both the drained and pristine plots. Depth of burn measurements and carbon emissions in the pristine plots are similar to measurements collected in other fires both in Canada and Alaska [30] , [31] , [32] . Hummock and hollow microforms in both the drained and pristine plots were present but were not pronounced, and our post-fire measurements represent an average of depth of burn across hummocks and hollows. Measurement of tree productivity and soil organic matter accumulation rates In 2003, we established replicate 10 m 2 plots in unburned pristine and drained portions of the fen. We selected five trees per plot to represent the full range in tree diameters present in each plot. A basal disk was collected from each tree and brought back to the laboratory. Each disk was sanded and scanned at high resolution, and ring-width measurements were determined using WinDendro software. We collected multiple peat cores (10 cm diameter, 40 cm in length) from each plot; all peat cores were frozen until analysis. Cores were sectioned into 2- to 4-cm depth increments based on changes in soil horizon, and were air dried. In one core per plot, we identified a macrofossil (usually a moss fragment) from near the bottom of each core for radiocarbon dating [36] . This approach assumes that rates of organic matter accumulation in the peat cores were similar across plots before drainage. Macrofossils were processed at the 14 C laboratory of the U. S. Geological Survey in Reston, Virginia including an acid-alkali-acid treatment, and 14 C ages were determined by accelerator mass spectrometry 14 C dating at the Center for Accelerator Mass Spectrometry, Lawrence Livermore National Laboratory, Livermore, California. We oven-dried peat core depth increments at 60 °C to a constant mass, weighed them for bulk density determination, and then homogenized them before C/N analysis using a Costech elemental analyzer. Soil carbon accumulation rates are based on 14 C ages and depth measurements of carbon content obtained through the elemental and bulk density measurements. Measurement of ground fuel combustion In the burned portion of the fen, we established replicate 10 m 2 plots in pristine and drained areas. Depth of burn was quantified using adventitious roots as a marker for pre-fire organic soil depth following the methods outlined in Turetsky et al . [30] and Kasischke et al . [37] Carbon losses associated with burning were estimated using depth of burn values and estimates of cumulative carbon accumulation with depth in peat cores collected from the unburned plots. How to cite this article: Turetsky, M. R. et al . Experimental drying intensifies burning and carbon losses in a northern peatland. Nat. Commun. 2:514 doi: 10.1038/ncomms1523 (2011).